Resource heterogeneity can facilitate cooperation Although social structure is known to promote cooperation, by locally exposing selfish agents to their own deeds, studies to date assumed that all agents have access to the same level of resources. This is clearly unrealistic. Here we find that cooperation can be maintained when some agents have access to more resources than others. Cooperation can then emerge even in populations in which the temptation to defect is so strong that players would act fully selfishly if their resources were distributed uniformly. Resource heterogeneity can thus be crucial for the emergence and maintenance of cooperation. We also show that resource heterogeneity can hinder cooperation once the temptation to defect is significantly lowered. In all cases, the level of cooperation can be maximized by managing resource heterogeneity. The emergence of cooperation in human and animal societies continues to intrigue evolutionary biologists [1] and sociologists. The fundamental social dilemma underlying the tragedy of the commons [2] is described by the Public Good Game (PGG) [2] . In the PGG, each of the n players has a budget R 1 of resources, from which he or she can contribute to a common pool that promotes a public good. The pooled resources are multiplied by r (1< r ≤ n ) and are divided evenly among all players ( r thus measures the gains from promoting the public good). When the group consists only of two players ( n =2) and a player can either cooperate by investing all personal resources into the common pool, or defect by investing none, this yields the following payoffs, denoted in analogy with the Prisoner’s Dilemma (PD) [3] : T = R 1 + R 1 r /2, R = R 1 r , P = R 1 and S = R 1 r /2. After rescaling (by setting the baseline and unit of payoffs to R 1 r /2) and substituting r =2/ b , this gives T=b , R= 1, P = b −1 and S =0, which is a special case (sometimes called ‘additive’) of the payoff structure of the PD [4] . Here the temptation to defect is measured by b −1; even though the players are always best-off collectively when they cooperate, if b >1 then an individual player will obtain a higher payoff by not contributing, no matter what the other players do. Therefore, defection is the evolutionarily stable strategy in this game. Although the PGG and PD illustrate that cooperators are prone to exploitation and that adaptation will favour free riders, ample examples of altruistic behaviour exist in human societies [5] and among other organisms [6] , [7] . To overcome this incongruity, the simple PGG model can be extended and made more realistic in a variety of ways. For example, repeated interactions and conditional strategies [8] , voluntary participation [9] , costly punishment of defectors [10] , confinement to groups [11] and elevated mortality of defectors under adverse environmental conditions [12] , [13] , have all been shown to facilitate the spread and maintenance of cooperators. Furthermore, embedding the cooperation game in ecological interactions may enable individuals to escape the dilemma [14] , [15] . Another notable extension situates players in physical space or on a social network; in such structured populations, cooperators can spread and persist if the temptation to defect is not too large [4] , [16] , [17] , [18] . The reason is that local interactions cause defectors to suffer from their own deeds; they can locally spread by exploiting cooperators, but then end up mostly interacting with other defectors, which drastically reduces the advantages of defection. Conversely, cooperators will mostly interact with other cooperators, which increase their payoff. Recently, interaction topologies other than regular graphs have been explored [19] , and it was shown that heterogeneous degree distributions facilitate the spread of cooperators [20] . Interestingly, previous analyses of the PGG always assumed that all players in a locale have access to the same level of resources. Therefore, the implications for cooperation of heterogeneity in the resource access, or wealth, of players have so far remained unexplored. For example, articles in a recent special issue in the Journal of Theoretical Biology devoted to cooperation studies do not touch this subject [21] . Although the effect of diversity in social structure [22] and of temporally variable resource availability for an entire population [23] are discussed, the fundamental question of how the diversity of resource availabilities within a population affects the level of cooperation has not yet been addressed. As uneven distributions of resources or wealth are ubiquitous, and as resource heterogeneity has already been shown to have an effect in a model of mutualism [24] between two different species, there is every reason to examine how evolutionarily stable levels of cooperation are influenced by resource heterogeneity. The notion of pooling and dividing resources in the PGG naturally generalizes to heterogeneous environments. We assume that each player has access to an amount of either R 1 or R 2 of resources (with R 2 > R 1 ). Depending on a player’s strategy, these resources can be either pooled (cooperator) or retained (defector). As before, the pooled resources are multiplied by r , with each participating player receiving half of the result. Only two parameters suffice to characterize this game (for details, see the derivation of the payoff matrix in the Methods section): b =2/ r (1< b <2) and c= ( R 2 − R 1 )/ R 1 , with b −1 measuring, as before, the temptation to defect and c measuring the wealth contrast between players on rich and poor sites. We consider a population of interacting and competing players that is spatially distributed on a square lattice, with rich and poor sites allocated at random and the fraction of rich sites given by p ; players interact with their four nearest neighbours (other interaction structures are also explored). We show that cooperation can be facilitated when some agents have access to more resources than others. Cooperation can then emerge even in populations in which the temptation to defect is so strong that agents would act selfishly if their resource access were uniform. However, resource heterogeneity can also hinder cooperation once the temptation to defect is significantly lowered. Our results thus demonstrate how managing resource heterogeneity can be crucial for safeguarding the emergence and maintenance of cooperation. At high temptation, heterogeneity facilitates cooperation Our results show that given the same high level of temptation to defect (corresponding to relatively low gains from promoting the public good), cooperators persist in the heterogeneous environment ( Fig. 1b ) even if they would go extinct in a homogeneous environment ( b −1>0.25) (ref. 25 , Fig. 1a ). In fact, a little bit of heterogeneity goes a long way towards stabilizing cooperation ( Fig. 2a,c,d ). 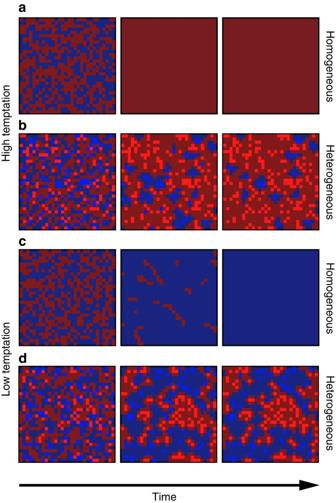Figure 1: Snapshots of the spatial configurations of cooperators and defectors. A 30 × 30 snapshot of spatial configurations of cooperators (blue) and defectors (red) of the 100 × 100 field in the spatial two-person PGG with (b,d) and without (a,c) wealth inequality, with rich sites indicated with brighter colours. Site qualities and initial strategies are set independently and at random, with (a,c) ap=0 and (b,d)p=0.2 fraction of rich sites and a 0.5 fraction of cooperators. Portraying the homogeneous environment as uniformly rich (p=1) or poor (p=0) is equivalent and can be used interchangeably. The initial distribution of strategies quickly changes within 106steps (middle column), but equilibrium is reached only after about 5 × 107steps (b–d, right column). When the temptation to defect is high (b−1=0.7;a,b), cooperation cannot be maintained in the homogeneous environment (a), whereas it persist in the heterogeneous environment (b). Note that clusters of cooperators always harbour a rich cooperator at their core (b). When the temptation to defect is low (b−1=0.1,c,d), defectors cannot survive in the homogeneous environment (c), but they cannot be ousted from the population in the heterogeneous environment (d). Note that rich defectors at the core of clusters make it possible for defection to be maintained (d). Other parameters:c=10 andm=10. Figure 1: Snapshots of the spatial configurations of cooperators and defectors. A 30 × 30 snapshot of spatial configurations of cooperators (blue) and defectors (red) of the 100 × 100 field in the spatial two-person PGG with ( b , d ) and without ( a , c ) wealth inequality, with rich sites indicated with brighter colours. Site qualities and initial strategies are set independently and at random, with ( a , c ) a p =0 and ( b , d ) p =0.2 fraction of rich sites and a 0.5 fraction of cooperators. Portraying the homogeneous environment as uniformly rich ( p =1) or poor ( p =0) is equivalent and can be used interchangeably. The initial distribution of strategies quickly changes within 10 6 steps (middle column), but equilibrium is reached only after about 5 × 10 7 steps ( b – d , right column). When the temptation to defect is high ( b −1=0.7; a , b ), cooperation cannot be maintained in the homogeneous environment ( a ), whereas it persist in the heterogeneous environment ( b ). Note that clusters of cooperators always harbour a rich cooperator at their core ( b ). When the temptation to defect is low ( b −1=0.1, c , d ), defectors cannot survive in the homogeneous environment ( c ), but they cannot be ousted from the population in the heterogeneous environment ( d ). Note that rich defectors at the core of clusters make it possible for defection to be maintained ( d ). Other parameters: c =10 and m =10. 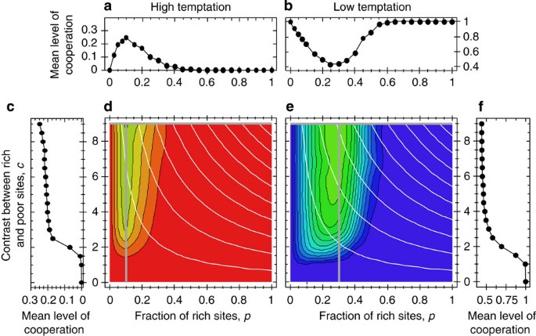Figure 2: Fraction of cooperators in heterogeneous environments. Equilibrium fractions of cooperators are shown as a function of the fractionpof rich sites and the contrastcbetween rich and poor sites. Panelsaandbshow mean levels of cooperation as a function ofpof rich sites atc=9. Panelscandfshow mean levels of cooperation as a function of the contrastcbetween rich and poor sites atp=0.1. Panelsa–candfshow transect of the parameter space explored in panelsdande, where the location of these transects is indicated by grey lines. Panelsdandedepict the fraction of cooperators through colour scales from 0 (red) to 1 (blue), based on 10 (a,c,d) or 40 (b,e,f) replicate model runs at each point, with increments of 0.1 inpand of 1 inc. White lines represent iso-wealth curves; along these, the average resource level of sites,pR2+(1−p)R1, remains constant. Initial strategies are set at random, with a 0.5 fraction of cooperators. Results are recorded after 5 × 108steps. Other parameters:m=10 andb−1=0.7 (high temptation:a,c,d) orb−1=0.1 (low temptation;b,e,f). Full size image Figure 2: Fraction of cooperators in heterogeneous environments. Equilibrium fractions of cooperators are shown as a function of the fraction p of rich sites and the contrast c between rich and poor sites. Panels a and b show mean levels of cooperation as a function of p of rich sites at c =9. Panels c and f show mean levels of cooperation as a function of the contrast c between rich and poor sites at p =0.1. Panels a – c and f show transect of the parameter space explored in panels d and e , where the location of these transects is indicated by grey lines. Panels d and e depict the fraction of cooperators through colour scales from 0 (red) to 1 (blue), based on 10 ( a , c , d ) or 40 ( b , e , f ) replicate model runs at each point, with increments of 0.1 in p and of 1 in c . White lines represent iso-wealth curves; along these, the average resource level of sites, pR 2 +(1− p ) R 1 , remains constant. Initial strategies are set at random, with a 0.5 fraction of cooperators. Results are recorded after 5 × 10 8 steps. Other parameters: m =10 and b −1=0.7 (high temptation: a , c , d ) or b −1=0.1 (low temptation; b , e , f ). Full size image Although a quantitative analytical theory of this spatial game seems beyond reach, some important qualitative insights can nevertheless be secured through a combination of numerical and analytical examinations. For this purpose, we quantify the most important departures between an observed spatial pattern and the corresponding mean-field pattern (with the latter defined by the random redistribution of site qualities and strategies). Important departures are those that are not only large, but also prevalent; we measure this by what we call the prevalent-deviation score (PDS) f log 10 ( f / ) calculated from a configuration’s observed frequency f and mean-field frequency . By observing the frequencies of every configuration of strategies and site qualities involving two to five players, and by determining the resultant PDS values ( Supplementary Note 1 ), we reveal the common characteristics of configurations that are prevalent and strongly deviate from mean-field expectations ( Fig. 3 ). 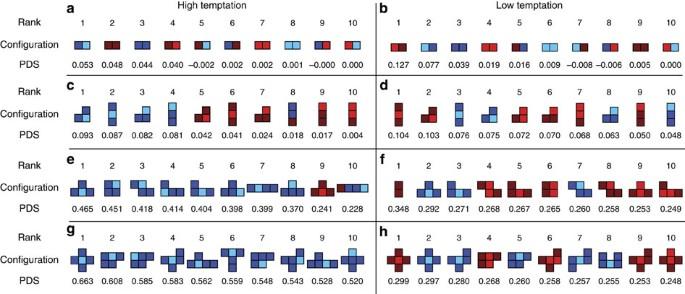Figure 3: Configurations with the highest prevalent-deviation score in heterogenous environment. First ten highest-ranking configurations are shown for (a,b) two, (c,d) three, (e,f) four and (g,h) five players. The model is first run for 5 × 107steps, after which configurations are recorded every 5 × 106steps for a total of 20 recordings. Frequencies belonging to mirror-symmetric and rotationally symmetric configurations are averaged and reported for one configuration arbitrarily chosen from the symmetry class. Colour coding as inFig. 1. Other parameters:m=10 andb−1=0.7,p=0.1,c=20 (high temptation;a,c,e,g) orb−1=0.1,p=0.3,c=6.67 (low temptation,b,d,f,h). Figure 3: Configurations with the highest prevalent-deviation score in heterogenous environment. First ten highest-ranking configurations are shown for ( a , b ) two, ( c , d ) three, ( e , f ) four and ( g , h ) five players. The model is first run for 5 × 10 7 steps, after which configurations are recorded every 5 × 10 6 steps for a total of 20 recordings. Frequencies belonging to mirror-symmetric and rotationally symmetric configurations are averaged and reported for one configuration arbitrarily chosen from the symmetry class. Colour coding as in Fig. 1 . Other parameters: m =10 and b −1=0.7, p =0.1, c =20 (high temptation; a , c , e , g ) or b −1=0.1, p =0.3, c =6.67 (low temptation, b , d , f , h ). Full size image At high temptation to defect, a rich cooperator is always found at the core of a cooperating cluster ( Figs 1b and 3a,b ). In the star-shaped configuration that has the highest PDS ( Fig. 3b ), if c /4> b −1 the poor-site cooperators have higher payoffs than any surrounding poor-site defector, whereas in a homogeneous environment ( c =0) this condition is never met for b −1>0. Hence, cooperators on rich sites enhance the payoffs of neighbouring cooperators on poor sites, and thus allow cooperation to spread in a heterogeneous environment. Our PDS analysis in Fig. 3a,b thus suggests that cooperators holding on to small rich islands are the main mechanism through which resource heterogeneity facilitates the maintenance of cooperation. This also explains why the highest facilitation of cooperative behaviour occurs at low values of p ( Fig. 2a,d ): under those conditions, rich islands are small, and, thus, are likely to harbour only cooperators, whereas the large, rich islands occurring when p is high are likely to harbour both cooperators and defectors, and consequently are easily taken over by defectors. At low temptation, heterogeneity hinders cooperation When the temptation to defect is low (corresponding to relatively high gains from promoting the public good), wealth inequality can lower cooperation levels ( Fig. 2e ) compared with a homogeneous environment. A low, but not vanishing fraction p of rich sites ( Fig. 2b,e ) and a high contrast c exacerbate this reduction in cooperation ( Fig. 2e,f ). Again, the five-site configuration with the highest PDS is star-shaped but now comprise poor-site defectors, with a rich-site defector at the centre ( Fig. 3d ). The rich site stabilizes the others if c >1.75/ b −1. Even for low temptations, 0< b −1<0.25, this inequality can be satisfied already at low contrast, for c >0.4 to c >0.75. As for high temptation, the occupancy of small, rich islands is important ( Figs 1b and 3c,d ); now, defectors can cling to these, but are ousted from larger ones. Analytical results obtained by investigating the dynamics of small clusters [25] corroborate the numerical result, by demonstrating how such clusters ( Supplementary Figs S1 and S2 ) behave differently in homogeneous versus heterogeneous environments ( Supplementary Note 2 ). Results are robust to alternate model assumptions The above results prove to be very robust. Changing the update rule (considering synchronous and/or deterministic updating instead of the asynchronous stochastic updating employed for the main figures) does not affect our qualitative results ( Supplementary Fig. S3 ). With deterministic updating, cooperators, at high temptation to defect, achieve slightly higher abundance than with stochastic updating ( Supplementary Fig. S3a ). This is in agreement with other theoretical investigations of cooperation in structured populations [17] . At low temptation to defect, the prevalence of defectors is much higher than with stochastic updating ( Supplementary Fig. S3b ). This is because a single defector amidst cooperators always has a higher payoff than its neighbours, so the defector can always spread. With stochastic updating, a single defector can go extinct just by chance. This explains why full cooperation cannot be achieved with deterministic updating ( Supplementary Fig. S3b,f ), but readily results for stochastic updating ( Fig. 2e and Supplementary Fig. S3d ). Introduction of non-overlapping generations (synchronous updating) causes no significant quantitative deviation from the results obtained for overlapping generations (asynchronous updating; compare Fig. 2d,e with Supplementary Fig. S3c,d , and Supplementary Fig. S3e,f with Supplementary Fig. S3a,b ). Considering the Moore neighbourhood (eight neighbours), a random regular network or a scale-free network result in the same qualitative outcomes ( Supplementary Fig. S4 ). The impact of the enlarged (Moore) neighbourhood is small. The level of cooperation increases in the heterogeneous high-temptation environment, when the interactions take place on a random regular graph. In other words, the randomization of neighbours further increases the effect of heterogeneity, so that for high temptation even higher levels of cooperation are achieved ( Supplementary Fig. S4c,d ). In contrast, the heterogeneous degree distribution of the scale-free interaction graph favours defection in heterogeneous environments ( Supplementary Fig. S4e,f ). Therefore, the levels of cooperation achieved in the heterogeneous high-temptation environment are more modest compared with those observed on regular lattices, and the drop in the levels of cooperation in the heterogeneous low-temptation environment is larger. Moreover, the possibility of erroneous execution of strategies does not affect the qualitative outcomes ( Supplementary Fig. S5 ). We can thus conclude that the noise introduced by such errors does not have any qualitative effects. When both strategies can err, the quantitative results hardly change for high temptation ( Supplementary Fig. S5a ), whereas the negative effects of environmental heterogeneity are enhanced when the temptation to defect is low ( Supplementary Fig. S5b ). At intermediate frequencies of rich sites, erring defectors can reap a high payoff by mistakenly cooperating if there are enough cooperators around. Such players, however, would still spread their defecting strategy. When only cooperators can err, the abundance of defectors is roughly the same for low temptation as in the absence of errors ( Supplementary Fig. S5d ). Cooperators, however, are generally better off if they can occasionally reap the benefit of defecting, while still propagating their cooperative behaviour ( Supplementary Fig. S5c ). Considering continuous resource levels does not even discernibly change our quantitative results ( Supplementary Fig. S6 ). The noise introduced by continuous resource levels has negligible effect on the outcome, showing that our assumption of only two resource levels does not affect the generality of the reported results. As a further test of robustness, we analyse the heterogeneous PGG for n =5 players, again finding qualitatively equivalent behaviour ( Supplementary Fig. S7 ). Moreover, when we replace the PD with the Snowdrift Game [26] , [27] , an important alternative for modelling cooperation, we find that resource heterogeneity always favours cooperation ( Supplementary Fig. S8 ). In summary, we have shown that our results are robust to a wide variety of changes in key features of our model ( Supplementary Table S1 ). Cooperation can emerge from scratch Our results show that cooperation can be maintained in a heterogeneous environment when this is impossible in the corresponding homogeneous environment. So far, however, we have assumed that players either always cooperate or always defect. In an attempt to encompass more real-world complexity, we now extend our model by allowing gradual evolution in the individual-level probability of players to cooperate. We can thus show that cooperation is not only maintained, but can also emerge from scratch through gradual evolution in heterogeneous environments initially comprising only defectors ( Fig. 4a ). In this mixed-strategy model of gradual evolution, the population-level averages of the probability to cooperate turn out to be closely similar to the frequencies of cooperators observed in the simpler, pure-strategy model (compare Fig. 2d,e with Fig. 4a,e , respectively). 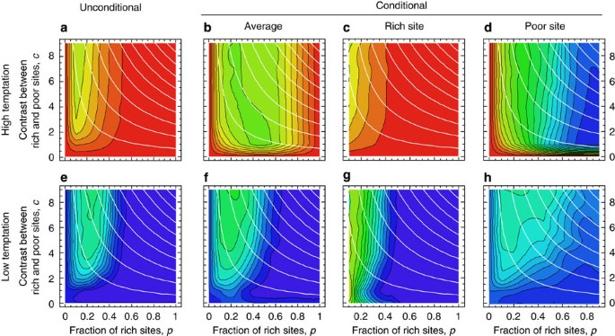Figure 4: Evolved propensities to cooperate in heterogeneous environment. Average equilibrium probabilities to cooperate are shown as a function of the fractionpof rich sites and the contrastcbetween rich and poor sites. Panelsaandeshow the evolutionary outcomes for unconditional strategies, whereas panelsb–dandf–hshow those outcomes for conditional strategies. In the latter case, the probabilities to cooperate when situated on a rich or poor site evolve independently. Average equilibrium probabilities to cooperate are shown in panelsbandf. The mean equilibrium probabilities of cooperation of players on rich sites are shown on panelscandg, and the same for players on poor sites in panelsdandh. All panels depict the fraction of cooperators through colour scales from 0 (red) to 1 (blue), based on five replicate model runs at each point, with increments of 0.1 inpand of 1 inc. Initial strategies were set to 0, implying defection on both rich and poor sites. As inFig. 2, white lines represent iso-wealth curves. Results are recorded after 2 × 109steps. Other parameters:m=10 andb−1=0.7 (high temptation;a,c,d) orb−1=0.1 (low temptation;b,e,f). Figure 4: Evolved propensities to cooperate in heterogeneous environment. Average equilibrium probabilities to cooperate are shown as a function of the fraction p of rich sites and the contrast c between rich and poor sites. Panels a and e show the evolutionary outcomes for unconditional strategies, whereas panels b – d and f – h show those outcomes for conditional strategies. In the latter case, the probabilities to cooperate when situated on a rich or poor site evolve independently. Average equilibrium probabilities to cooperate are shown in panels b and f . The mean equilibrium probabilities of cooperation of players on rich sites are shown on panels c and g , and the same for players on poor sites in panels d and h . All panels depict the fraction of cooperators through colour scales from 0 (red) to 1 (blue), based on five replicate model runs at each point, with increments of 0.1 in p and of 1 in c . Initial strategies were set to 0, implying defection on both rich and poor sites. As in Fig. 2 , white lines represent iso-wealth curves. Results are recorded after 2 × 10 9 steps. Other parameters: m =10 and b −1=0.7 (high temptation; a , c , d ) or b −1=0.1 (low temptation; b , e , f ). Full size image These results can be understood by appreciating that the cooperative act is an investment towards the objective of being surrounded by cooperators. Players on rich sites can maintain this cooperative neighbourhood by being cooperative themselves, up to the point at which the resultant advantage is balanced by the danger of facilitating invasion by a less cooperative player residing on an adjacent rich site. In a further extension, we analyse the evolution of conditional strategies, with each player now being characterized by two continuous variables: the probability to cooperate if the player is on a rich site, and the probability to cooperate if the player is on a poor site. Allowing conditional strategies to evolve results in amplified effects of heterogeneity. With conditional strategies, only a little contrast between rich and poor sites ( c =1) already suffices for the population to reap the full benefit of wealth inequality through increased cooperation ( Fig. 4b ). Moreover, the range of fraction p of rich sites over which heterogeneity enables cooperation is considerably broadened relative to the unconditional case ( Fig. 4b ). Remarkably, players evolve a higher probability to cooperate when situated on poor sites than when residing on rich sites (compare Fig. 3c,d ), with the probability to cooperate on rich sites increasing, as rich sites become scarce. Note that when there are very few rich sites, the players on these sites are more inclined to cooperate and the resultant average level of cooperation is mainly due to their contributions (compare Fig. 4c,d ). At low levels of temptation, populations cease to exhibit full cooperation when poor sites abound, and this departure grows as wealth inequality increases ( Fig. 4f ). In this case, players on rich sites are reluctant to cooperate when their numbers are low, as exploitation of their altruistic behaviour leads to elevated defection. Consequently, the probability of players on rich sites to cooperate steadily increases with their abundance ( Fig. 4g ). In general, players on poor sites tend to be more cooperative than players on rich sites. This is because a group of poor-site players can increase their payoffs more if they become more cooperative, whereas a group of rich-site players can maintain their competitive superiority even with a more modest cooperativeness. Resource heterogeneity allows cooperation to persist even when the temptation to defect is so high that full defection is observed in the homogeneous case. This key finding of our study is broadly related to an earlier research, demonstrating that asymmetries among players can facilitate the spread of cooperation. Maynard Smith [28] , for instance, showed that role asymmetry through the introduction of the ‘bourgeois’ strategy can lessen aggression in the Hawk–Dove Game. Moreover, variation in the total number of interaction links individuals possess on heterogeneous interaction graphs results in elevated levels of cooperation [20] , [29] . This is because some individuals can then reap benefits from many interactions, resulting in inequalities in the maximal benefits of players [30] . Similarly, the existence of role models (individuals whose successes are copied more often than those of others) can stabilize cooperation [31] , [32] , but see Kim et al. [33] Thus, differences among individuals appear to be an important, and as yet insufficiently studied, determinant of the cooperation level a society can attain. Interpreting our results in a wider context, it is tempting to ask whether they might contribute an explanatory facet to the scientific understanding of more or less egalitarian social norms [34] . Our results suggest that the level of cooperation can be managed by changing the distribution of wealth (moving along the iso-wealth curves in Figs 2 and 3 ). Although differences among individuals are pervasive in the living world and in human societies, social norms can either counter or exacerbate them. Specifically, in situations in which the temptation to defect is high (as gains from promoting the public good are low), it will always be possible to increase the levels of cooperation by increasing wealth inequality ( Figs 2d and 3a,b ). On the other hand, in situations in which gains from promoting the public good are high (and the temptation to defect thus is low), wealth inequalities lead to decreased levels of cooperation ( Figs 2e and 3e,f ). In the latter case, the evolution of inequality aversion, promoting an egalitarian society, can considerably increase levels of cooperation by decreasing wealth inequalities, ultimately leading to a situation in which all members of a population receive the same share of resources. Egalitarian motives in humans are widespread and are exhibited from a very early age [35] , [36] , [37] . Fehr and Schmidt [38] have thus suggested equity as a key factor in strengthening human cooperation and in explaining the prevalence of cooperation in our species [34] , [39] . The case for animals having inequality aversion is less strong. Some studies have documented strong reactions by animals towards what they perceive as inequity [40] , [41] , [42] , [43] ; yet, the larger shares accrued by socially dominant individuals are seldom questioned by other individuals [41] and the resultant social disapproval is even less strong towards members of the same social group [42] . On the other hand, some studies found that great apes are true rational maximizers when it comes to their feeding options [44] , [45] and no inequality aversion could be found among them. If we account for the facts that great apes and humans both exhibit cooperative behaviour [46] , but human cooperation is much more pervasive [47] and efficient at generating public goods, we can arrive at the conclusion that (early) humans and great apes are positioned on opposite sides of the threshold in the efficiency of public-good generation; below this threshold heterogeneity and inequity are beneficial, whereas above this threshold homogeneity and equity should be the norm ( Fig. 2d,e ). Examples for such disparate efficiencies abound, for example, chimpanzees, can cooperatively hunt only small monkeys [48] , whereas human hunters can take down large preys [49] ; likewise, chimpanzees physically attack only lonely individuals from other bands, whereas humans regularly engage in warfare [50] . This suggests that cooperation was a necessity in the evolutionary past of our species, and that the efficiency of our cooperation has co-evolved with our egalitarian motives. Although humans appear to have been fully egalitarian at the hunter–gatherer stage of cultural evolution [51] , and although contemporary hunter–gatherer societies still exhibit low levels of wealth inequality [52] , industrial and post-industrial societies have varied levels of wealth inequality [53] and also show variation in the level of observable cooperative tendencies [54] , [55] , [56] . This suggests that our results might help explain the re-emergence of inequality during the Holocene [57] . As human societies became larger, and mechanisms limited to enabling the maintenance of cooperation in small-scale societies (like peer reputation and peer punishment [55] ) thus lost their effectiveness, institutions emerged that allowed enforcing cooperative norms at a cost [58] , [59] . Maintaining the same level of cooperation at the lower efficiency implied by the involved cost required elevated wealth inequality, which indeed prevailed for hundreds of years [57] . Today we hopefully are in the middle of a new transition in the cultural evolution of our species, back to more egalitarian societies. Indeed, modern Western societies exhibit high levels of cooperativeness [56] coupled with low wealth inequalities comparable to those of the hunter–gatherers [52] . Our model-based analyses suggest that this transition could have come about by an increased effectiveness of public-good generation. Egalitarianism, a unique human trait, can once more hold sway in our societies. Payoff matrix The payoff matrix ( Table 1 ) is obtained in four steps. First, players on a poor site can invest R 1 , whereas players on a rich site can invest R 2 ; cooperators invest, whereas defectors do not. The pooled investments are multiplied by r and then evenly distributed among the two players. Second, payoffs are normalized by adjusting the payoff baseline so that a cooperator on a poor site playing against a defector on a poor site receives a payoff of 0. Third, payoffs are normalized by adjusting the payoff unit, so that two cooperators on poor sites playing against each other will each receive a payoff of 1. These two normalizations have no bearing on game dynamics. Fourth, the definitions b =2/ r and c =( R 2 − R 1 )/ R 1 are applied to arrive at the payoff matrix shown below. Note that switching cooperation to defection in this matrix always increases a player’s payoff by b −1 on a poor site and by ( c+ 1)( b −1) on a rich site, irrespective of the partner’s strategy or site quality. Note also that the site quality of partners affects a player’s payoff only when their partners cooperate, but not when they defect. Table 1 Payoff matrix of the two-person Public Good Game with wealth inequality. Full size table Game dynamics Our spatial game dynamics are analogous to those analysed, for example, by Nowak et al. [4] Individual players reside on sites of a 100 × 100 square lattice with periodic boundary conditions. Updating is asynchronous, by randomly choosing a focal site to be updated in each step. The player on this focal site then plays the game described in the main text with all four nearest neighbours, and these neighbours in turn play it with their four nearest neighbours. The focal site is held by the focal player, or is taken over by its neighbours, with probabilities proportional to their payoffs raised to the power of m (resulting in what is known as proportional or imitation updating [27] ), which thus characterizes the degree of stochasticity in the contest for a site [4] . When a site’s occupancy changes, the payoffs of the focal player and its neighbours are updated. Evolutionary dynamics In our evolutionary analysis, the game dynamics are as described above, except that the lattice size is reduced to 64 × 64 sites to keep computation time manageable. Each player’s strategy is given by his or her probability to cooperate in an interaction. If a site’s occupancy changes, there is a 5% chance that the focal player’s strategy is mutated. The mutated strategy is chosen randomly from the interval [ x −0.05, x +0.05], where x is the strategy before mutation, and any mutated strategy outside the interval [0,1] is reset to the corresponding boundary. Evolutionary dynamics start with every player being a defector, implying a vanishing probability to cooperate. We also allow strategies to be conditional on the quality of the occupied site, resulting in two cooperation probabilities that can evolve independently. Upon mutation, one of these two probabilities is chosen at random and is changed as described above. Robustness checks Many alternate model assumptions are examined. With asynchronous deterministic updating, the player with the highest payoff always wins the local competition, which is equivalent to m →∞. This update rule is called ‘best takes over’ [26] . With synchronous stochastic updating, all players’ payoffs and strategies are updated at the same time. This corresponds to the dynamics of a population with non-overlapping generations. In practice, synchronous updating is carried out by determining the outcome of competition based on the state of a site at time t , and continuing with the winners of all corresponding local competitions at time t +1. With synchronous deterministic updating, the player with the highest payoff always wins the local competition and all players’ payoffs and strategies are updated at the same time. In the model variant in which the interaction structure is described by the Moore neighbourhood, each player plays with its eight neighbours, which include the four orthogonal and the four diagonal neighbours. In the case when interactions take place on a random regular graph, the neighbourhood relations are fully randomized at the beginning of each model run. This means that each player has k =4 neighbours, but these players can be located anywhere on the original lattice. The scale-free graphs are generated by the Albert–Barabási method [60] at the beginning of each model run. In this case, on average, each player has k =4 neighbours, but the actual numbers of neighbours follow a power-law distribution. Payoffs are scaled to the actual number of neighbours before comparing them in competition. Erroneous strategy execution is modelled as follows: in each individual game, each player has a small probability ( ε =0.01) accidentally to play the opposite strategy (that is, cooperators defect, whereas defectors cooperate). Of course, such an event only affects strategy execution at one moment but never lastingly changes the strategy itself. As a further test, we examine what happens if defectors would not, by mistake, behave as cooperators. We, therefore, also consider a setup in which cooperators can erroneously defect, whereas defectors never cooperate. As players in our model do not base their behaviours on the behaviours perceived in their neighbours, erroneous perception need not be considered. Continuous levels of resources are incorporated by considering a continuous bimodal distribution of resources instead of just two discrete levels of resources. Specifically, resources are either low, R 1 + ρ , or high, R 2 + ρ , where ρ is a random number drawn from a Gaussian distribution with mean 0 and s.d. σ . Payoffs are calculated by pooling the available resources from cooperators, dividing by b =2/ r (see the payoff matrix section of the Methods), and giving the result to both participant of the game. Defectors withhold their resources. In the heterogeneous Snowdrift Game, each player can gain a benefit from cooperation, b 1 on rich sites or b 2 on poor sites (with b 1 > b 2 ), and the cost of cooperation is c 0 for any player. In the Snowdrift Game, the cost is halved when both players cooperate, and the benefit is reaped when at least one of the players cooperates. We use synchronous stochastic updating, as described above. The five-player PGG is a generalization of the two-player PGG, in which a player and N −1 of its neighbours constitute a group playing a round of the PGG. As in the basic game, players on poor sites can invest R 1 , whereas players on rich sites can invest R 2 ; cooperators invest, whereas defectors do not. The pooled investments are multiplied by r and are then evenly distributed among the N players. After applying the definition of contrast, c =( R 2 − R 1 )/ R 1 , and normalizing payoffs by R 1 , we obtain the payoff of a cooperator as Π= r ( k poor +( c +1) k rich )/ N , where k poor and k rich are the numbers of cooperators within the group situated on poor and rich sites, respectively. Analogously, the payoff of a defector is Π+1 on a poor site and Π+( c +1) on a rich site. How to cite this article: Kun, Á. and Dieckmann U. Resource heterogeneity can facilitate cooperation. Nat. Commun. 4:2453 doi: 10.1038/ncomms3453 (2013).